Nuclear retention of the transcription factor NLP7 orchestrates the early response to nitrate in plants Nitrate is both an important nutrient and a signalling molecule for plants. Although several components of the nitrate signalling pathway have been identified, their hierarchical organization remains unclear. Here we show that the localization of NLP7, a member of the RWP-RK transcription factor family, is regulated by nitrate via a nuclear retention mechanism. Genome-wide analyses revealed that NLP7 binds and modulates a majority of known nitrate signalling and assimilation genes. Our findings indicate that plants, like fungi and mammals, rely on similar nuclear retention mechanisms to instantaneously respond to the availability of key nutrients. Nitrogen (N), which is an essential macronutrient for living organisms, enters the food chain mainly through the assimilation performed by higher plants. Plant growth and crop productivity often are limited by low N availability in the soil. Therefore, nitrate has an important role in plant growth and development [1] . In addition to its role as a major nutrient for plants, nitrate acts as an important signalling molecule for several developmental processes such as root growth or flowering [2] . Indeed, nitrate controls the expression of over a thousand genes [3] , [4] ; however, the molecular players involved in this signalling pathway are largely unknown [5] . Indeed, only a few transcription factors (ANR1, NLP7, LBD37/38/39, SPL9 (refs 6 , 7 , 8 , 9 )) implicated in the regulation of gene expression by nitrate have been identified, and most of these factors are encoded by genes that are themselves regulated by nitrate at the transcriptional level. One exception is NIN-Like Protein7 (NLP7), a putative transcription factor that is expressed constitutively and shares homology with NIN (for Nodule INception), an essential protein for nodulation in legumes [10] . Molecular and physiological analyses suggest that NLP7 is involved in plant responses to nitrate [7] . Here we show that, on nitrate supply, NLP7 is retained inside the nucleus to coordinate an early response to the availability of this essential nutrient. Nitrate triggers the nuclear accumulation of NLP7 To investigate if NLP7 itself is regulated by nitrate supply, we expressed a fully functional pNLP7:NLP7–GFP fusion construct ( Supplementary Fig. S1 ) in the nlp7-1 Arabidopsis mutant and examined the subcellular localization of this NLP7 fusion in response to nitrate. Whereas NLP7–GFP was mostly localized in the nucleus in the presence of nitrate ( Fig. 1a ), it was detected only in the cytoplasm after N-starvation ( Fig. 1b ). Resupplying nitrate after N-starvation led, within minutes, to the relocation of NLP7–GFP into the nucleus ( Fig. 1c , Supplementary Fig. S2 and Supplementary Movie 1 ). This relocalization was promoter independent as it occurred regardless of whether NLP7–GFP expression was driven by the constitutive CaMV 35S promoter or the native NLP7 promoter ( Supplementary Fig. S3 ). Furthermore, this nuclear accumulation was rapidly reversible when nitrate was withdrawn ( Fig. 1e–h , Supplementary Fig. S3e–h ). Finally, this rapid nuclear relocation was specific to nitrate and independent of the counter cations K + or NH 4 + as other N sources did not trigger nuclear translocation of NLP7–GFP ( Supplementary Figs. S4 and S5 ). Based on these observations, we conclude that nitrate itself triggers the rapid relocation of NLP7 into the nucleus. 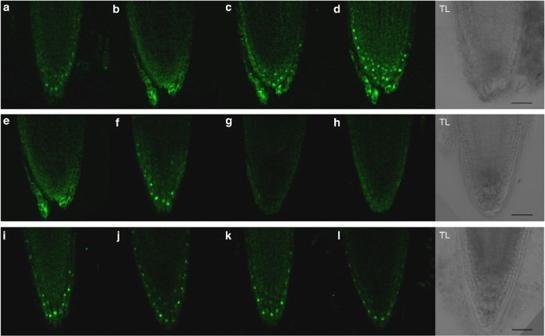Figure 1: Nucleocytosolic shuttling of NLP7 is regulated by nitrate. Confocal imaging was performed onnlp7-1seedlings expressing pNLP7-driven NLP7–GFP fusion protein. (a) Seedlings grown on nitrate. (b–d) Nitrate addition kinetics: N-starved seedlings (b) were transferred to a nitrate medium and observed after 3 (c) and 6 min (d). (e–h) Nitrate depletion kinetics: N-starved seedlings (e) were transferred to a nitrate medium for 20 min (f), then to N-free medium and observed after 10 (g) and 20 min (h). (i–l) Effect of leptomycin B (LMB) on the subcellular location of NLP7–GFP on nitrate addition and depletion. N-starved seedlings were incubated with LMB in a N-free medium for 3 h (i), then transferred for 20 min to nitrate medium (j) and thereafter depletion kinetics were recorded after 10 (k) or 20 min (l). Bright field images are shown for each time series (TL, transmitted light), the length of the scale bar corresponds to 50 μm. Figure 1: Nucleocytosolic shuttling of NLP7 is regulated by nitrate. Confocal imaging was performed on nlp7-1 seedlings expressing pNLP7-driven NLP7–GFP fusion protein. ( a ) Seedlings grown on nitrate. ( b – d ) Nitrate addition kinetics: N-starved seedlings ( b ) were transferred to a nitrate medium and observed after 3 ( c ) and 6 min ( d ). ( e – h ) Nitrate depletion kinetics: N-starved seedlings ( e ) were transferred to a nitrate medium for 20 min ( f ), then to N-free medium and observed after 10 ( g ) and 20 min ( h ). ( i – l ) Effect of leptomycin B (LMB) on the subcellular location of NLP7–GFP on nitrate addition and depletion. N-starved seedlings were incubated with LMB in a N-free medium for 3 h ( i ), then transferred for 20 min to nitrate medium ( j ) and thereafter depletion kinetics were recorded after 10 ( k ) or 20 min ( l ). Bright field images are shown for each time series (TL, transmitted light), the length of the scale bar corresponds to 50 μm. Full size image NLP7 localization is regulated by nitrate-dependent nuclear retention The presence of a predicted leucine-rich nuclear export signal within NLP7 ( Supplementary Fig. S6 ) prompted us to test if the cytoplasmic localization of NLP7 during nitrate starvation could result from its nuclear export by the Exportin1 CRM1/XPO1 ( [11] , [12] ). In N-starved NLP7–GFP seedlings that had been treated for 3 h with leptomycin B (LMB), an inhibitor of Exportin1 ( [13] ), NLP7–GFP exhibited partial nuclear accumulation ( Fig. 1i , Supplementary Fig. S3i ). This nuclear retention is consistent with the hypothesis that NLP7 is exported actively from the nucleus in the absence of nitrate rather than imported actively into the nucleus in the presence of nitrate. Also supporting active nuclear export, LMB treatment inhibited the rapid translocation of NLP7–GFP from the nucleus to the cytoplasm when nitrate-grown seedlings were shifted to N-starvation ( Fig. 1j–l , Supplementary Fig. S3j–l ). Taken together, these data highlight the exquisite regulation of NLP7 subcellular location in response to nitrate availability. NLP7 binds hundreds of genes including many genes involved in nitrate signalling and assimilation Because NLP7 is a putative transcription factor, we sought to identify the genomic regions bound by NLP7 on its nitrate-induced relocation into the nucleus. Instead of using artificial, inducible nuclear localization methods, we took advantage of the rapid and specific nuclear relocalization of NLP7 that is induced by nitrate and subsequently identified NLP7-bound DNA regions. To this end, N-starved seedlings expressing pNLP7:NLP7–GFP in the nlp7-1 mutant background were resupplied with nitrate for 10 min before crosslinking and chromatin immunoprecipitation (ChIP) with an anti-GFP antibody of the NLP7-bound chromatin fragments ( Supplementary Fig. S7 ). By hybridizing the immunoprecipitated DNA to a whole-genome tiling array (ChIP-chip [14] ), we identified 851 genes bound by NLP7 in the presence of nitrate ( Supplementary Data 1 ). Gene Ontology (GO) term analysis revealed a significant enrichment for genes involved in N-metabolism and related metabolic pathways, such as the oxidative pentose–phosphate (OPP) pathway, sulphur- and carbon-metabolism, as well as genes involved in hormone metabolism and in transport ( Fig. 2a ). Moreover, among the bound genes were nearly all of those previously characterized as being involved in nitrate signalling, such as ANR1 (ref. 6 ), LBD37/38 (ref. 8 ), CIPK8 (ref. 15 ) and NRT1.1 (refs 16 , 17 ; Supplementary Table S1 ). As expected for a transcription factor, NLP7 binding was localized preferentially near the transcriptional start site of its target genes ( Fig. 2b ). Indeed, 511 out of the 851 gene sequences bound by NLP7 corresponded to 5′promoter regions. However, no enriched DNA-binding motifs were found among the NLP7-immunoprecipitated sequences. For example, the NRE (nitrate response element) consensus sequence that was identified in the NiR promoter [18] was not detected by pattern searching (RSAT tools [19] ). Quantitative ChIP-PCR analysis was used to validate the NLP7 binding to four genes, NRT2.1, NRT2.2, NIA1 and LBD37, all of which are regulated by nitrate ( Fig. 2c ). In the case of NIA1 , NLP7 binding was also detected downstream of the gene, consistent with the requirement of additional 3′ end sequences for the proper induction of this gene by nitrate [20] . To directly test the effect of NLP7 on its bound genes, transient transactivation assays were performed in Arabidopsis protoplasts using the reporter construct pNRT2.1:LUC, which contains the luciferase gene under the control of the NRT2.1 promoter [21] and includes the sequence bound by NLP7. Co-transformation of pNRT2.1:LUC with p35S:NLP7 increased the luciferase activity sevenfold compared with the control pNRT2.1:LUC without p35S:NLP7 ( Fig. 2e ). Taken together, these results show that NLP7 is a bona fide transcription factor that likely acts as a master regulator of the early response to nitrate. 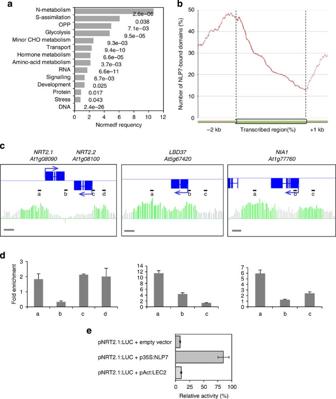Figure 2: Genome-wide NLP7 binding in response to nitrate. (a) Gene ontology (GO) term enrichment for the high confidence NLP7 target genes. GO terms were defined using Mapman bins and sorted on frequency related toArabidopsisset. AssociatedP-values of the hypergeometric distribution are indicated, which were calculated as follows:P=BC(M,x) × BC(N−M,n−x)/BC(N,n). BC is the binomial coefficient, calculated as follows: BC(n, k)=n!/(k! × [n−k]!). In the above equations,xis the number of input genes with the selected classification,nis the total number of input genes,Mis the number of genes with the selected classification in the database (MapMan) andNis the total number of genes in this database. (b) Spatial distribution and number of NLP7-bound domains in proximity to transcribed regions. To account for different gene size, the positions of binding sites within transcribed regions were calculated relative to their length. (c,d) ChIP-chip and ChIP-qPCR data at selected NLP7 target genes. (c) The exon–intron structure and orientation of target genes are shown in the top half of each panel. NLP7 ChIP-chip profile is shown at the bottom half; probes reporting a significant enrichment of NLP7 binding in response to nitrate are indicated in green. Amplicons analysed indare given as black line and numbered a–d. Scale bar, 1 kb. (d) Real-time ChIP-PCR at selected targets on an independent biological replicate. Position of amplified fragments is indicated inc. Each PCR amplification of the immunoprecipitated samples was normalized to the respective input. The fold enrichment of the nitrate-induced NLP7 binding was calculated as the ratio between the +nitrate and the –N immunoprecipitated amplification signals. (e) Transactivation of pNRT2.1:LUC by NLP7. After co-transfection of pNRT2.1:LUC, p35S:NLP7 and p35S:GUS inArabidopsisprotoplasts, luciferase activity was measured relative to p35S:GUS activity. pACT:LEC2 was used as a control transcription factor. Figure 2: Genome-wide NLP7 binding in response to nitrate. ( a ) Gene ontology (GO) term enrichment for the high confidence NLP7 target genes. GO terms were defined using Mapman bins and sorted on frequency related to Arabidopsis set. Associated P -values of the hypergeometric distribution are indicated, which were calculated as follows: P =BC( M , x ) × BC( N−M , n − x )/BC( N , n ). BC is the binomial coefficient, calculated as follows: BC( n, k )= n !/( k ! × [ n − k ]!). In the above equations, x is the number of input genes with the selected classification, n is the total number of input genes, M is the number of genes with the selected classification in the database (MapMan) and N is the total number of genes in this database. ( b ) Spatial distribution and number of NLP7-bound domains in proximity to transcribed regions. To account for different gene size, the positions of binding sites within transcribed regions were calculated relative to their length. ( c , d ) ChIP-chip and ChIP-qPCR data at selected NLP7 target genes. ( c ) The exon–intron structure and orientation of target genes are shown in the top half of each panel. NLP7 ChIP-chip profile is shown at the bottom half; probes reporting a significant enrichment of NLP7 binding in response to nitrate are indicated in green. Amplicons analysed in d are given as black line and numbered a–d. Scale bar, 1 kb. ( d ) Real-time ChIP-PCR at selected targets on an independent biological replicate. Position of amplified fragments is indicated in c . Each PCR amplification of the immunoprecipitated samples was normalized to the respective input. The fold enrichment of the nitrate-induced NLP7 binding was calculated as the ratio between the +nitrate and the –N immunoprecipitated amplification signals. ( e ) Transactivation of pNRT2.1:LUC by NLP7. After co-transfection of pNRT2.1:LUC, p35S:NLP7 and p35S:GUS in Arabidopsis protoplasts, luciferase activity was measured relative to p35S:GUS activity. pACT:LEC2 was used as a control transcription factor. Full size image NLP7 broadly impacts the rapid regulation of gene expression by nitrate To further assess the role of NLP7 in the early response to nitrate, we profiled, genome wide, the transcripts of wild type (wt) and two allelic loss-of-function nlp7 mutant plants during a short-term nitrate-resupply kinetics and compared their respective nitrate response transcriptomic profiles ( Fig. 3a , Supplementary Data 2 ). We found that 25% of the genes in the wt that were differentially regulated after a 10 min nitrate supply following N-starvation showed a weaker or an opposite response in at least one of the two nlp7 mutants log (2) expression ratios either ≥0.5 or ≤−0.5, 176 out of 712 genes, Supplementary Data 3 ). Moreover, after 10 and 20 min of nitrate induction, the fraction of genes that was deregulated in at least one of the nlp7 mutants increased to 58% (383 out of 661 genes, Supplementary Data 4 ). These results indicate that NLP7 has a profound and broad influence on the early transcriptome response to nitrate. 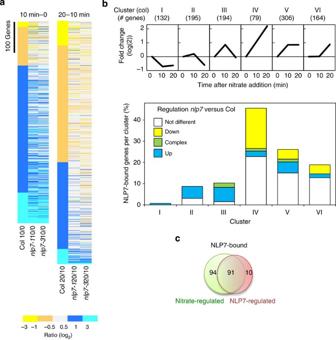Figure 3: NLP7-binding and direct regulation of nitrate-regulated gene clusters. (a) Differential expression of genes in nitrate-induced wt (Col) andnlp7mutants. N-starved seedlings were exposed to nitrate for 10 or 20 min and transcriptome variations were analysed using CATMA arrays. Differentially expressed genes (log(2)expression ratios either >0.5 or < −0.5) were ordered from the lowest to the highest ratio using the wt (Col) comparisons as reference. The corresponding ratios in nitrate response ofnlp7mutants are shown for each gene (0, 10, 20: time in minutes after nitrate supply). (b) Distribution of NLP7-bound genes within nitrate-regulated gene clusters. Top panel, six gene clusters (I–VI) were defined based on the expression pattern observed in the wt after nitrate supply. The numbers of genes in each cluster as well as their average expression trend (black line) are given. Bottom panel, distribution of NLP7-bound genes in the different clusters according to their regulation by nitrate in thenlp7mutants in comparison to the wt: down (yellow), up (blue), not different (white). Complex (green) stands for a mixed up/down pattern at the two time points (10 and 20 min). (c) Venn diagram showing the number of NLP7-bound genes that are differentially expressed innlp7mutants (red circle) and NLP7-bound genes that are regulated by nitrate (green circle). Figure 3: NLP7-binding and direct regulation of nitrate-regulated gene clusters. ( a ) Differential expression of genes in nitrate-induced wt (Col) and nlp7 mutants. N-starved seedlings were exposed to nitrate for 10 or 20 min and transcriptome variations were analysed using CATMA arrays. Differentially expressed genes (log (2) expression ratios either >0.5 or < −0.5) were ordered from the lowest to the highest ratio using the wt (Col) comparisons as reference. The corresponding ratios in nitrate response of nlp7 mutants are shown for each gene (0, 10, 20: time in minutes after nitrate supply). ( b ) Distribution of NLP7-bound genes within nitrate-regulated gene clusters. Top panel, six gene clusters (I–VI) were defined based on the expression pattern observed in the wt after nitrate supply. The numbers of genes in each cluster as well as their average expression trend (black line) are given. Bottom panel, distribution of NLP7-bound genes in the different clusters according to their regulation by nitrate in the nlp7 mutants in comparison to the wt: down (yellow), up (blue), not different (white). Complex (green) stands for a mixed up/down pattern at the two time points (10 and 20 min). ( c ) Venn diagram showing the number of NLP7-bound genes that are differentially expressed in nlp7 mutants (red circle) and NLP7-bound genes that are regulated by nitrate (green circle). Full size image NLP7 binding leads to both activation and repression of nitrate-responsive genes To clearly distinguish between direct and indirect effects, we determined whether the genes that showed a modified nitrate response in the nlp7 mutants were bound by NLP7. In total, we identified 91 genes that both exhibited an altered expression in the nlp7 mutants in response to the nitrate signal and were bound by NLP7. Among these direct targets of NLP7 were nearly proportionate numbers of genes that were either less induced or less repressed by nitrate in the nlp7 mutants compared to wt ( Supplementary Data 5 ). Whether NLP7 activates or represses a target gene presumably is determined by the structure of the promoter, the binding sites, the flanking sequences and the interplay with other transcriptional regulators as previously observed [22] , [23] . To deepen this analysis, we clustered the nitrate-responsive genes according to their expression pattern in wt plants ( Fig. 3b , Supplementary Fig. S8 and Supplementary Data 6 ). In the highly nitrate-inducible cluster IV, 36 out of 79 genes were bound by NLP7, representing the highest proportion of bound genes among the clusters. Almost half of these 79 genes showed modified nitrate response kinetics in the nlp7 mutants, with mainly a decreased induction compared with the wt, indicating that NLP7 is an activator of these nitrate-induced genes ( Fig. 3b , Supplementary Data 7 ). For clusters V and VI, which correspond to nitrate induction between 0 and 10 min and between 10 and 20 min, respectively, one-third of the NLP7-bound genes showed modified nitrate response kinetics in the nlp7 mutants. Within the nitrate-repressed or transiently induced genes (clusters I, II and III) the majority of the few NLP7-bound genes (<10%) in these clusters were upregulated in the nlp7 mutants compared with the wt ( Fig. 3b , Supplementary Data 7 ), suggesting that, in these cases, NLP7-dependent nitrate repression was impaired. NLP7 directly regulates different steps of N assimilation The most highly enriched GO terms among the direct NLP7 targets that both are detected by ChIP-chip and less nitrate-induced in nlp7 mutants are N assimilation and the OPP pathway ( Supplementary Fig. S9 ). The OPP pathway is a critical step providing reductants for nitrate assimilation and has been shown to have a very early response to nitrate resupply [9] . Accordingly, the list of NLP7-dependent nitrate-inducible genes includes nitrate transporter NRT2.1 , nitrate reductase NIA1 , nitrite reductase, glutamine synthetase 2, uroporphyrinogen III methyltransferase 1, ferredoxin 3 and transketolase (At3g60750) ( Fig. 4a , Supplementary Fig. S10 and Supplementary Data 7 ). In addition, putative new regulatory proteins involved in the early nitrate signalling were identified within the NLP7 targets such as MAPKKK13 (MEKK13), bHLH34 and NLP3 ( Fig. 4b , Supplementary Fig. S11 and Supplementary Data 7 ). 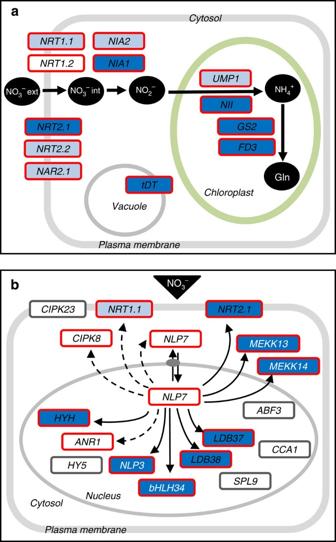Figure 4: NLP7 directly regulates many steps of the primary N assimilation and nitrate signalling pathways. (a) N assimilation pathway from nitrate uptake on the plasma membrane to ammonium incorporation into C-skeletons. Depicted is a plant cell, with plasma membrane, cytosol, chloroplast and vacuole.NRT, nitrate transporter;NAR2, nitrate-assimilation-related 2 (NRT3.1);NIA, nitrate reductase;NII, nitrite reductase;UMP1,S-adenosyl-L-methionine-dependent uroporphyrinogen III methyltransferase 1;GS2, glutamine synthetase;GOGAT, glutamine-oxoglutarate-aminotransferase (GLU1, GLU2, GLS);tTD, tonoplastic malate/fumarate transporter. (b) Nitrate signalling from nitrate perception by nitrate transceptors NRT1.1 and NRT2.1 to the regulation of gene expression. All known and several putative regulators (black and white writing, respectively) are depicted in a plant cell with plasma membrane, cytosol and nucleus.NRT, nitrate transporter/nitrate sensor;CIPK, calcineurin B-like (CBL)-interacting protein kinase;MEKK, mitogen-activated kinase kinase kinase;HY5,long hypocotyl5; HYH,HY5 homologue;ANR1, Arabidopsis nitrate regulated 1;bHLH, basic helix-loop-helix transcription factor;LBD, lateral organ boundary domain;ABF3, auxin-binding factor 3;CCA1, circadian clock associated 1;SPL9, squamosa promoter binding protein-like 9. The colour of the border of each gene represents the results from the ChIP-chip experiment: genes with a red border are bound by NLP7, genes with a grey border are not bound by NLP7. Dark and light blue represent the results from expression profiling during nitrate addition kinetics; light blue: gene was induced by nitrate, dark blue: gene was induced by nitrate and less nitrate-regulated in thenlp7mutants. Black letters: genes already characterized, white letters, newly identified gene as putatively involved in nitrate signalling. All gene products might not occur in the same cell type. Figure 4: NLP7 directly regulates many steps of the primary N assimilation and nitrate signalling pathways. ( a ) N assimilation pathway from nitrate uptake on the plasma membrane to ammonium incorporation into C-skeletons. Depicted is a plant cell, with plasma membrane, cytosol, chloroplast and vacuole. NRT , nitrate transporter; NAR2 , nitrate-assimilation-related 2 ( NRT3.1 ); NIA , nitrate reductase; NII , nitrite reductase; UMP1 , S -adenosyl- L -methionine-dependent uroporphyrinogen III methyltransferase 1; GS2 , glutamine synthetase; GOGAT , glutamine-oxoglutarate-aminotransferase (GLU1, GLU2, GLS); tTD , tonoplastic malate/fumarate transporter. ( b ) Nitrate signalling from nitrate perception by nitrate transceptors NRT1.1 and NRT2.1 to the regulation of gene expression. All known and several putative regulators (black and white writing, respectively) are depicted in a plant cell with plasma membrane, cytosol and nucleus. NRT , nitrate transporter/nitrate sensor; CIPK , calcineurin B-like (CBL)-interacting protein kinase; MEKK , mitogen-activated kinase kinase kinase; HY5, long hypocotyl5 ; HYH, HY5 homologue; ANR1 , Arabidopsis nitrate regulated 1; bHLH , basic helix-loop-helix transcription factor; LBD , lateral organ boundary domain; ABF3 , auxin-binding factor 3; CCA1 , circadian clock associated 1; SPL9 , squamosa promoter binding protein-like 9. The colour of the border of each gene represents the results from the ChIP-chip experiment: genes with a red border are bound by NLP7, genes with a grey border are not bound by NLP7. Dark and light blue represent the results from expression profiling during nitrate addition kinetics; light blue: gene was induced by nitrate, dark blue: gene was induced by nitrate and less nitrate-regulated in the nlp7 mutants. Black letters: genes already characterized, white letters, newly identified gene as putatively involved in nitrate signalling. All gene products might not occur in the same cell type. Full size image We confirmed the modified nitrate-responsive expression pattern of these genes by quantitative reverse transcription-PCR ( Supplementary Figs S10 and S11 ). This highly sensitive detection method allowed us to show that several of the lowly expressed genes bound by NLP7, for which no differential expression between nlp7 mutants and wt was detected in our microarray analyses, were indeed differentially regulated by nitrate in the nlp7 mutant background. This was the case for the LBD37 , LBD38, MAPKKK14 ( MEKK14 ) and HYH genes ( Supplementary Fig. S11 ). NLP7 binds to nitrate-responsive genes A large fraction of the NLP7-bound genes was not differentially expressed in the nlp7 mutants compared to the wt during the early response to nitrate. This result is not surprising as binding of a given transcription factor, as detected by ChIP-chip, does not necessarily correlate with effective transcription modulation of the corresponding gene by the same factor [24] . The action of transcription factors is modulated by the genomic landscape of DNA regulatory sequences and co-regulatory proteins. In addition, some of the NLP7-bound genes have very low expression levels, and, thus, the microarray analysis might have failed to determine their expression differences, such as was the case for LBD37 , LBD38, MAPKKK14 ( MEKK14 ) and HYH . In addition, some of the NLP7 targets may require longer periods of nitrate induction to show significant expression changes. It is also possible that some targets may be regulated by NLP7 only after accumulation of a cofactor not present in our experimental condition or may be expressed in specific cells or developmental stages excluded from our study. Indeed, in addition to the 91 NLP7-bound genes that are deregulated for early nitrate response in the nlp7 mutants, there are 94 NLP7-bound genes that are regulated by nitrate during our short nitrate supply kinetic, but do not show a differential response in the nlp7 mutant ( Fig. 3c , Supplementary Data 8 ). For these genes, deregulated expression in the mutants might have been missed in our experimental conditions. In total, the percentage of nitrate-regulated genes among the NLP7-bound genes is four times higher than the genome-wide 3.8% of nitrate-regulated genes in our short-term nitrate supply experiment. It is important to note that among the NLP7-bound and differentially expressed genes in the nlp7 mutants, only a small fraction (10 out of 101) corresponds to genes that are not regulated by nitrate ( Fig. 3c , Supplementary Table S2 ), pointing clearly to the fact that NLP7 is primarily implicated in nitrate signalling. We showed here that the transcription factor NLP7 is a main regulator of nitrate signalling. The intracellular localization of NLP7 is specifically and rapidly regulated by nitrate and mediated by a nuclear retention mechanism. In plants, nucleocytosolic shuttling is a major regulatory mechanism involved, for example, in the signalling cascades triggered by light, by brassinosteroids or plant pathogen interaction [25] . However, no such mechanism has been identified for nutrient signalling in plants so far. Our data indicate that the nuclear export of NLP7 slows down within minutes after the addition of nitrate, allowing a rapid NLP7-dependent regulation of gene expression. Consistent with our data, Krouk et al . [9] showed that gene expression is regulated by nitrate as rapidly as 2 min after supply. Our work identifies direct NLP7 target genes. Through ChIP-chip we identified 851 NLP7-bound genes only after a 10 min-response to nitrate. Consistent with the role of NLP7 in nitrate response, NLP7-bound genes are highly enriched for regulatory and structural genes of nitrate metabolism and signalling. NLP7-bound domains possess an average size of 1,114 bp (with a mean size of 859 bp). However, pattern searching did not detect any significant consensus motifs among the NLP7-bound fragments. Previous searches for nitrate-responsive elements have been conducted, but, with the exception of the NRE, which is involved in nitrate regulation of NiR (ref. 18 ), no such elements have been identified so far. We did not find enrichment of the NRE sequence among the NLP7-bound fragments. Moreover, Chlamydomonas NIT2, a RWP-RK protein related to NLP7, also has been shown to bind sequences unrelated to NRE elements [26] , indicating that the RWP-RK proteins are not likely candidates for NRE-binding proteins. Our ChIP-chip analysis together with our genome-wide analysis of nitrate-regulated gene expression in nlp7 mutants under the same experimental conditions, allowed us to identify direct target genes of NLP7. We showed that the loss of NLP7 leads to a sizeable rearrangement of the transcriptional response to nitrate, impacting the expression of genes involved in both nitrate signalling and assimilation. Moreover, NLP7 was shown to act as both a transcriptional activator and a repressor depending possibly on its regulatory partners. Our rather stringent approach likely underestimated the number of genes that are regulated directly by NLP7 in response to nitrate due to, on the one hand, the low expression of putative target genes, and on the other hand, to possible redundant regulation by other transcription factors, such as other NLPs. Indeed, the sequence of NLP6 is highly homologous to NLP7. Thus, it is possible that NLP6 and other NLPs could bind some NLP7 targets and regulate their expression in the absence of NLP7. However, the fact that the nlp7 mutants, but not other nlp mutants, have a clear nitrate-related phenotype [7] supports the hypothesis that NLP7 is the major regulatory element among NLP proteins. Together, the overlap between NLP7-bound genes and deregulated gene expression in nlp7 mutants highlighted a subset of genes mainly related to nitrate assimilation and oxidative pentose pathway, suggesting that NLP7 is one of the master regulators of nitrate signalling. However, a significant fraction of the nitrate-regulated genes were not bound by NLP7. These genes may either be regulated by other signalling pathways or be indirectly controlled by NLP7 through NLP7-dependent regulators. Indeed, the fact that NLP7 loss-of-function does not totally abolish the responses to nitrate ( Supplementary Fig. S1 ) indicates that NLP7-independent nitrate signalling cascades likely exist. Consistent with this observation, four other NLP genes have been identified as direct targets of NLP7 (NLP1, NLP2, NLP3 and NLP5; Supplementary Table S1 ). Our data indicates that the hypothesis that tight regulation between NLP proteins controls nitrate signalling needs to be challenged. The deregulation of direct NLP7 targets has far-reaching consequences for genome-wide nitrate regulation. Indeed, the transcriptomic changes that result from NLP7 loss-of-function extend beyond the genes directly bound by NLP7. Secondary effects arising from the loss-of-function of NLP7 are larger ( Supplementary Fig. S8 ) than changes of transcript abundance for NLP7-bound genes. These indirect target genes might be under the control of additional regulatory circuits, as regulatory protein-encoding genes are themselves bound and transcriptionally regulated by NLP7. Thus, a small deregulation of a subset of genes targeted by NLP7 can have an expansive effect on nitrate-responsive genome-wide gene expression, pinpointing the upper hierarchical role of NLP7 as an orchestrator of nitrate responses. Taken together, the swift regulation of NLP7 by nitrate and the functional diversity of NLP7 target genes highlight the important and broad role of NLP7 in the plant primary nitrate response. Indeed, NLP7 regulates the expression of genes involved in a range of biological activities from nitrate transport and assimilation to transduction of the nitrate signal by various regulators. This coordinated regulation by NLP7 ensures rapid adaptation to N availability to maintain plant nitrate homeostasis. Unlike most signalling molecules, nitrate is also a main nutrient for plants. In Saccharomyces species, nutrients have been shown to regulate the nuclear export of tRNAs [27] , [28] . Plants, like mammals, do not seem to directly regulate nuclear export of tRNA in response to nutrient stress [29] . So far, nutrient-dependent regulation of the nuclear export of transcription factors has been shown for NirA, the master regulator of N assimilation in the filamentous fungus Aspergillus [30] , and for FoxO1, a Forkhead box transcription factor involved in the regulation of metabolism in mammals [31] . Therefore, our finding that nuclear export of NLP7 is regulated by nitrate suggests convergent evolution in distant organisms of mechanisms that enable instant responses to the availability of key nutrients. Plant material and culture conditions The two nlp7 allelic knockout mutants, nlp7-1 and nlp7-3, were in the Columbia (Col-8) wt background of Arabidopsis thaliana . The nlp7-1 mutant background was used for complementation by the pNLP7:NLP7–GFP or by p35S:NLP7–GFP constructs [7] . Plants were grown on a 3 mM KNO 3 liquid medium (3 mM KNO 3 , 1 mM KH 2 PO 4 /K 2 HPO 4 , 0.5 mM CaSO 4 , 0.5 mM MgCl 2 , 3 mM MES, pH 5.8, 0.25% (w/v) sucrose, supplemented with microelements (modified from (ref. 4 )) in long-day photoperiod (16/8 h at 25 °C with 80 μmol photons.m −2 s −1 ). Confocal imaging Plants were grown for 5 days on the 3 mM KNO 3 liquid medium (see above), nitrogen-starved for 2 days by exchanging the culture medium with a nitrogen-free medium, in which KNO 3 was replaced by KCl. Plants were mounted in 40 μl of a top agar (0.1%, w/v) solution. During confocal imaging, either 5 μl of 0.5 M KNO 3 , 5 μl of 0.5 M NH 4 Cl, 2.5 μl of 0.5 M NH 4 NO 3, 15 μl of 50 mM glutamine or 5 μl of 0.5 M KNO 2 were added to the mounting medium; the same plantlets were imaged during a time course. For nitrate depletion, plantlets were grown as described above, then transferred for 20 min to 3 mM nitrate medium, and finally transferred to N-free medium. At each time point of the kinetics, a new plantlet was withdrawn from the medium for immediate imaging. For the nuclear export inhibition experiment, a 3-h preincubation with LMB (Sigma, at 100 nM final concentration) was performed in the N-free medium. LMB was then added at each step. Laser scanning confocal imaging was performed using the Zeiss 710 microscope equipped with an argon laser (488 nm for green fluorescent protein (GFP) excitation). Emission was collected at 510 to 545 nm (GFP). The images were coded green for GFP. For nuclei staining, plantlets were stained with 4′, 6-diamidino-2-phenylindole (DAPI, 5 μg ml −1 ; Invitrogen). The excitation wavelength was 405 nm and the emission was collected at 420–480 nm. A sequential scanning mode was used when DAPI marker staining was combined with GFP to minimize the crosstalk between the two partially overlapping emission spectra. The images were coded green (GFP) and red (DAPI) giving yellow co-localization in merged images. Images were processed in ImageJ and Photoshop Element (Adobe Systems). Chromatin immunoprecipitation Seedlings were grown for 10 days on a 3 mM KNO 3 liquid medium. Plants were then nitrogen-starved for 3 days by changing the culture medium with a nitrogen-free medium, in which KNO 3 was replaced by KCl. A 10-min nitrate induction was performed by changing the culture medium for the 3 mM nitrate solution (+N). For the control samples (−N), the nitrogen-free solution was changed for a fresh one. ChIP was performed essentially, as described in Gendrel et al ., [32] using 3.5 μl of anti-GFP antibody and Dynabeads coupled with Protein A and G (Invitrogen). Reverse crosslinking was carried out with the iPure kit (Diagenode). Immunoprecipitated DNA was amplified using the Whole Genome Amplification 4 kit (Sigma), differentially labelled and co-hybridized in dye-swap experiments according to the manufacturer’s instructions (Roche NimbleGen). ChIP-chip analysis of NLP7 binding regions was performed in two biological replicates (two-dye swaps). ChIP-chip analysis Hybridization data were normalized using an analysis of variance model to remove technical biases. Data were averaged on the dye-swap to remove tile-specific dye biases and across biological replicates. Normalized data were then analysed using a three-states Parsimonious Higher-Order Hidden Markov Model (PHHMM, www.jstacs.de/index.php/PHHMM ) to model the joint distribution of the +N and−N-derived signals, taking into account spatial dependency between the DNA sequence reported by the probes on the tiling array [33] . Briefly, normalized log2 +N/−N signal ratio for each probe corresponds to the observed values of the Hidden Markov chain, while the hidden chain is the enrichment state of the DNA sequence reported by each probe in the ChIP-chip experiments, respectively. This PHHMM procedure was applied to the data following a two-step process. First, initial model parameters are iteratively maximized by a specific Bayesian Baum-Welch training algorithm enabling the integration of previous knowledge and by a data-dependent reduction of transition parameters. Second, based on this training, optimized model parameters are obtained that allow the parsimonious higher-order HMM with univariate Gaussian emission distributions to effectively model spatial dependencies between measurements [33] . This HMM approach provides a probabilistic classification of each probe into one of the three states, namely non-enriched, enriched and depleted in the +N/−N comparison. Adjacent probes belonging to the same HMM-derived state are joined into domains by requiring a minimal run of 400 bp and allowing a maximal gap of 200 bp. An enrichment probability is assigned to each domain by calculating the median probability of each probe within a domain. Data were deposited in Gene Expression Omnibus (GEO) under the accession number GSE36763 . ChIP-PCR The ChIP-chip data were validated by ChIP-quantitative PCR (qPCR), on the two hybridized biological replicates as well as on a third biological replicate. qPCR was performed using LightCycler-FastStart DNA Master SYBR Green I kit (Roche) according to the manufacturer’s protocol on a Eppendorf Realplex qPCR machine. Specific primer sets are given in Supplementary Table S3 . Each amplification of the immunoprecipitated samples was normalized to the respective input. The fold enrichment of the nitrate-induced NLP7 binding was calculated as the ratio between +N and the −N immunoprecipitated amplification signal. Transcriptome analysis Plantlets (Col-8, nlp7-1 and nlp7-3 mutants) were grown as described for ChIP. The whole plantlets were collected at time point 0 (before nitrate addition), 10 and 20 min after nitrate addition. Total RNA extractions from two independent biological replicates were performed using GenElute Mammalian Total RNA kit from Sigma-Aldrich, modified by adding a DNase step (Qiagen RNase-free DNase kit). Microarray analysis was carried out at the Research Unit in Plant Genomics in Evry, France, using the CATMA array (V5) containing 24,576 gene-specific tags corresponding to 22,089 genes from Arabidopsis [34] . The analysis was performed as in Lurin et al . [35] In short, cRNAs were produced from 2 μg of total RNA (Message Amp aRNA kit, Ambion). Then 5 μg of cRNAs were reverse transcribed in the presence of 300 units of SuperScript II (Invitrogen), cy3-dUTP, and cy5-dUTP (NEN), and purified and concentrated with YM30 Microcon columns (Millipore). Slides were prehybridized for 1 h and hybridized overnight at 42 °C in 25% formamide. After washing the arrays were scanned, and images were analysed by GenePix Pro 3.0 (Axon Instruments). For each comparison one technical replication with fluorochrome reversal was performed for each biological duplicate. For the wt (Col-8) transcriptome analysis, the following sample comparisons were performed in two biological replicates: Col 10 min vs Col T0; Col 20 min vs Col 10 min. For each mutant the following sample comparisons were done: nlp7 T0 vs Col T0; nlp7 10 min vs Col 10 min and nlp7 20 min vs Col 20 min. Analysis of transcriptome data Experiments were designed with the Bioinformatic and Predictive Genomics group at the Unité de Recherche en Génomique Végétale in Evry, France. Specific statistics were developed to analyse CATMA hybridizations. For each array, the raw data comprise the logarithm of median feature pixel intensity (in log base 2) at wavelengths of 635 nm (red) and 532 nm (green). No background was subtracted. An array-by-array normalization was performed to remove systematic biases as described before [35] . In short, after excluding bad spots, a global intensity-dependent normalization using the Loess procedure was performed to correct the dye bias, followed by a correction for print tip effects on each metablock. To determine differentially expressed genes, we performed a paired t- test on the log ratios averaged on the dye swap. A trimmed variance was calculated from spots that did not display extreme variance. The raw P- values were adjusted by the Bonferroni method, which controls the family-wise error rate (with a type I error equal to 5%). We also adjusted the raw P- values to control a false discovery rate using Benjamini-Yetkutieli at a level of 1%. In the CATMA analysis pipeline, family-wise error rate proved to be the best solution to balance the estimated number of false positives and false negatives [36] . As described before [37] , when the Bonferroni P- value was lower than 0.05, the gene was declared differentially expressed. Microarray data were deposited in GEO under the accession number GSE39261 . GO terms were defined using the classification superviewer tool at http://bar.utoronto.ca/ntools/cgi-bin/ntools_classification_superviewer.cgi using Mapman bins and sorted on frequency related to Arabidopsis set. Quantitative reverse transcription–PCR RNA was extracted with Trizol method (Invitrogen). First-strand cDNAs were synthesized using Moloney murine leukaemia virus reverse transcriptase and oligo(dT) 15 primers (Promega) [38] , [39] . PCR was performed as for ChIP-PCR. Specific primer sets are given in Supplementary Table S3 . Promoter transactivation in Arabidopsis protoplasts For promoter transactivation assays, Arabidopsis protoplasts were prepared from cell cultures by a sucrose gradient after 3 h of cell wall digestion as in Thomine et al . [39] polyethylene glycol (PEG)-mediated transfection was performed using 10 μg of plasmid DNA. Plasmids were obtained from M. Lepetit (pNRT2.1:LUC) [21] and from B. Dubreucq (pACT:LEC2) [40] . The p35S:NLP7 construct was obtained by subcloning into pBS [7] . Protoplasts were co-transfected with the p35S:GUS plasmid (pRTL2-GUS ( [41] )) as control. Eighteen hours after transfection, β-glucuronidase and luciferase activity were measured as described previously [42] , [43] . In short, protoplasts were extracted with a Triton X-100 containing buffer, and enzyme activities were measured using a fluorogenic or a light emitting assays with 4-methyl umbelliferyl glucuronide and luciferin, respectively, as substrate. Luciferase activity was expressed relative to p35S:GUS activity. How to cite this article: Marchive C. et al . Nuclear retention of the transcription factor NLP7 orchestrates the early response to nitrate in plants. Nat. Commun. 4:1713 doi: 10.1038/ncomms2650 (2013).